Quantum Faraday and Kerr rotations in graphene Graphene, a monolayer sheet of carbon atoms, exhibits intriguing electronic properties that arise from its massless Dirac dispersion of electrons. A striking example is the half-integer quantum Hall effect, which endorses the presence of Dirac cones or, equivalently, a non-zero (π) Berry’s (topological) phase. It is curious how these anomalous features of Dirac electrons would affect optical properties. Here we observe the quantum magneto-optical Faraday and Kerr effects in graphene in the terahertz frequency range. Our results detect the quantum plateaus in the Faraday and Kerr rotations at precisely the quantum Hall steps that hallmark the Dirac electrons, with the rotation angle defined by the fine-structure constant. The robust quantum Hall plateaus in the optical regime, besides being conceptually interesting, may open avenues for new graphene-based optoelectronic applications. Graphene offers a unique opportunity to study the physics of Dirac fermions in condensed matter [1] , [2] that arises from the low-energy band structure with a conical (massless Dirac) dispersion in the effective-mass approximation. The experimental fabrication of monolayer graphene [3] has instigated studies of various interesting properties that reflect the nature of massless Dirac fermions, where a notable example is the half-integer quantum Hall effect (QHE) characteristic of Dirac cones [4] , [5] , [6] , [7] . Although the quantum phenomena peculiar to graphene have been primarily observed in transport properties, it is gradually beginning to be recognized that the Dirac-fermion nature in graphene has profound effects on dynamical (optical) response, as exemplified by the universal light absorption π α ( α , the fine-structure constant) in the near-visible region [8] . The magneto-optical Faraday (Kerr) effect, in which linearly polarized light has its polarization plane rotated when transmitted through (reflected by) a material in the presence of a magnetic field or magnetization, can be thought of as the ‘optical-Hall effect’ when the phenomenon arises from conducting electrons. Then we can pose a question whether the QHE can be observed in the Faraday and Kerr rotations in graphene; this is a highly nontrivial question, as we do not know whether the degradation of the topological protection of the quantized dc Hall conductivity should entirely wash out the QHE phenomena in the ac regime. Physically, the integer QHE in the dc regime is intimately related to the carrier localization [9] , and how this can be extended to the optical regime is an intriguing question. Recently, a theoretical investigation has demonstrated the appearance of plateau-like structures in the optical Hall conductivity, which was predicted to be observable in Faraday rotation in the photon energy region as large as the cyclotron energy (that is, inter-Landau-level (LL) transitions) in a conventional nonrelativistic two-dimensional electron gas system [10] . Further, the effect has also been predicted for graphene, where the optical-Hall effect should reflect the peculiar QHE that arises from the massless Dirac dispersion in graphene [10] . The Faraday rotation has also been anticipated for the Dirac fermions in time-reversal symmetry broken topological insulators, as a consequence of magnetoelectric coupling, the effect of which can be implemented into the quantized surface Hall conductance [11] , [12] . Therefore, the Faraday effect in graphene provides an opportunity to test the anticipated optical-Hall effect of Dirac fermions in solids. Although the ac QHE has indeed been observed in a 2DEG in a GaAs heterostructure in the microwave [13] , [14] and recently in the quasi-optical (terahertz; THz) frequency [15] ranges, the Faraday effect in graphene, namely in a Dirac-electron system, in the QHE regime has remained elusive. With recent progress in the fabrication of large-area epitaxial graphene on SiC substrate, the measurement of the Faraday effect in monolayer graphene has been performed in the far-infrared region and been accounted for by the classical Drude model [16] . Here we observe the THz Faraday and Kerr rotations in monolayer graphene in the QHE regime. Faraday and Kerr rotations exhibit values defined by the fine-structure constant α ~1/137, as anticipated if one assumes the ac Hall conductivity has an overall value similar to the dc one. [17] The optical QHE in a one-atom-thick system, while conceptually interesting, is made conspicuous by the present finding that quantum Hall plateaus appearing in the magneto-optical response are anomalously robust in relatively low magnetic fields, which reflects graphene's large LL spacings that characterize the Dirac electron. Transport properties characterized by THz spectroscopy For the THz experiments, we have employed a large area (10 × 10 mm 2 ) monolayer graphene epitaxially grown on the Si face of SiC [18] , [19] , [20] . 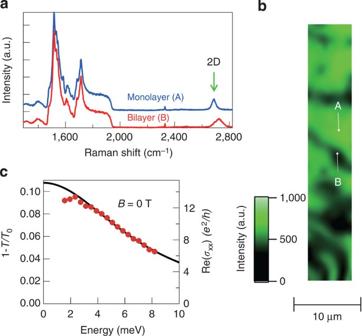Figure 1: Raman image of the graphene on SiC and the optical conductivity spectrum. (a) The 532 nm Raman spectra of the epitaxial graphene on the SiC substrate at the points A and B in the Raman imaging data of (b) taken at the 2D-band of monolayer graphene. The signals below 2,000 cm−1are mostly attributed to that from SiC substrate. (c) The absorption spectrum (left axis) and the optical conductivityσxx(ω) spectrum (right axis) of graphene in the THz range at zero magnetic field. A bare SiC substrate was used as a reference. The solid curve is the fitted result with the Drude model. Figure 1a shows the 532 nm Raman spectra exhibiting the 2D-band specific to the monolayer graphene [21] . The spatial mapping of this 2D-band in Fig. 1b indicates the growth of monolayer graphene with a micrometre scale uniformity (see the Methods section for details). Figure 1c shows the longitudinal optical conductivity spectrum σ xx ( ω ) of graphene averaged over the spot size of the THz beam (1.2 mm for 1 THz) obtained from the transmission-type THz time-domain spectroscopy (THz-TDS). All the THz measurements are performed at 5 K. The spectrum is well fitted by the Drude model, σ xx ( ω )= iD /π( ω + i Γ ), where Γ is the damping parameter and is the Drude weight with n being the carrier density and v F =1 × 10 6 m s −1 the Fermi velocity [22] , [23] . From the fit, the carrier density is estimated as n =2.2 × 10 11 cm −2 and the corresponding Fermi energy as | E F |=56 meV through the relation n = E F 2 / πħ 2 v F 2 . The mobility is estimated as μ = v F 2 e /| E F | Γ =2 × 10 4 cm 2 V −1 s −1 with Γ =7 meV. As the coverage of monolayer graphene in the sample is 80%, the Fermi energy estimated here is a value averaged over the spot size of the probe THz beam. Figure 1: Raman image of the graphene on SiC and the optical conductivity spectrum. ( a ) The 532 nm Raman spectra of the epitaxial graphene on the SiC substrate at the points A and B in the Raman imaging data of ( b ) taken at the 2D-band of monolayer graphene. The signals below 2,000 cm −1 are mostly attributed to that from SiC substrate. ( c ) The absorption spectrum (left axis) and the optical conductivity σ xx ( ω ) spectrum (right axis) of graphene in the THz range at zero magnetic field. A bare SiC substrate was used as a reference. The solid curve is the fitted result with the Drude model. 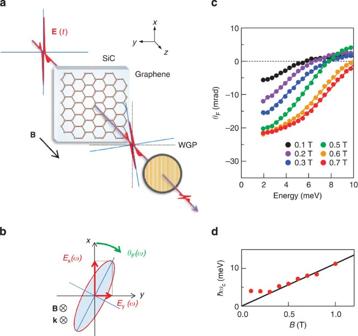Figure 2: Faraday rotation in the low magnetic field regime. (a) Schematic of the time-domain THz polarimetry. The incident THz pulse with the electric field (E-field) linearly polarized alongxdirection is irradiated onto the sample in a magnetic field (B//z). The Faraday effect induces the orthogonal (y-) component of the E-field of the transmitted pulse. A wire-grid polarizer (WGP) is placed beyond the sample to measure the parallel and orthogonal components of the transmitted THz E-field,Ex(t) andEy(t), respectively. (b) Definition of the Faraday rotation angleθF(ω). (c) The Faraday rotation spectra (circles) versus photon energy at 5 K in magnetic fields between 0.1 and 0.7 T. The solid curves are fitted by using the Drude model. (d) The cyclotron frequencies as a function of the magnetic field, obtained from the fitting in (c). The solid line is the calculated one withEF=60 meV. Full size image Magneto-optical Faraday effect Figure 2a depicts the schematic configuration for the Faraday rotation measurement with THz-TDS (see the Methods section for details). Figure 2b defines the sign of the rotation angle with respect to the direction of the magnetic field and the light propagation vector. Figure 2c shows the Faraday rotation θ F ( ω ) in a low magnetic field regime below 0.7 T. The magnitude of the Faraday rotation angle is seen to increase with the magnetic field, where the sign of the Faraday rotation in the low frequency limit indicates that the carriers are electrons. In the thin-film limit, the Faraday rotation angle is expressed as [24] Figure 2: Faraday rotation in the low magnetic field regime. ( a ) Schematic of the time-domain THz polarimetry. The incident THz pulse with the electric field (E-field) linearly polarized along x direction is irradiated onto the sample in a magnetic field ( B // z ). The Faraday effect induces the orthogonal ( y -) component of the E-field of the transmitted pulse. A wire-grid polarizer (WGP) is placed beyond the sample to measure the parallel and orthogonal components of the transmitted THz E-field, E x ( t ) and E y ( t ), respectively. ( b ) Definition of the Faraday rotation angle θ F ( ω ). ( c ) The Faraday rotation spectra (circles) versus photon energy at 5 K in magnetic fields between 0.1 and 0.7 T. The solid curves are fitted by using the Drude model. ( d ) The cyclotron frequencies as a function of the magnetic field, obtained from the fitting in ( c ). The solid line is the calculated one with E F =60 meV. Full size image where n sub (=3.1) is the refractive index of the substrate (SiC) [25] , Z 0 =377 Ω the vacuum impedance, σ ( ω )= σ xx ( ω )± iσ xy ( ω ) the optical conductivity for the right and left circularly polarized light. The Faraday rotation spectra in Fig. 2c are well fitted by the Drude model (solid curves), according to which the optical Hall conductivity is expressed as σ xy ( ω )= Dω c /π[( ω+iΓ ) 2 − ω c 2 ], where ω c = ev F 2 B /| E F | is the cyclotron frequency for graphene [22] . Here, we set D , Γ and ω c as fitting parameters, where D and ω c are not independent. The ω c obtained from the fit exhibits a linear dependence on the magnetic field above 0.4 T as shown in Fig. 2d , from whose slope the Fermi energy is estimated as E F =60 meV. This value is consistent with the Drude weight ( D ) and also with that obtained from the Drude fit to σ xx ( ω ) at zero field. The linear dependence of the cyclotron frequency indicates that the system is in the classical limit [22] . In low magnetic fields below 0.3 T, ω c obtained from the fit remains nearly constant, whereas the cyclotron resonance should vanish at zero magnetic field. Some excitations not taken into account in the Drude fit, plausibly magnetoplasmons where the cyclotron resonance is coupled with the plasmon localized in the step-and-terrace structure of epitaxial graphene [26] , may be contributing to the optical Hall conductivity spectrum in low magnetic fields. When we further increase the magnetic field above 1 T, the Faraday rotation turns to decrease as shown in Fig. 3a . Above 3 T the Faraday rotation becomes frequency-independent, where the cyclotron frequency stays far above the observation frequency. Notably, the rotation angle is pinned to a value of θ F =−5 mrad and hardly changes above 4 T, which is more clearly seen in the magnetic field dependence of the rotation angle at 4 meV (1 THz) ( Fig. 3b ). The dashed curve represents the classical Drude model as obtained to fit the data in the low magnetic field regime below 0.7 T with the parameters of E F =60 meV and Γ =7 meV. Here the calculated curve is multiplied by a factor of 0.7, which will be discussed later in detail. Although the Drude model well reproduces the data in the low-field regime, a clear deviation is discerned above 3 T as a shoulder structure. To indicate the magnetic field scale, the inset of Fig. 3b illustrates the LL energies in graphene, ( n =0, 1, 2, …) [6] . The first LL exceeds the Fermi energy of 60 meV at 3 T, above which the LL filling of ν =2 is realized. Therefore, the observed plateau structure in the Faraday rotation can be attributed to the ν =2 QHE. With the graphene QHE of σ xy =− νe 2 / h =−2(2 n +1) e 2 / h for ν =2, the Faraday rotation angle is anticipated to take a value θ F =−4 α /(1+ n sub )=−7.1 mrad, as given by equation (1) neglecting the term Re( Z 0 σ ± ) (<<1+ n sub ). This value is close to the observed −5 mrad in the plateau region. 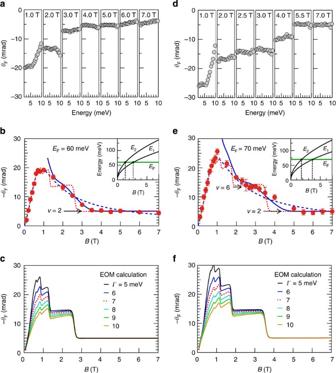Figure 3: Faraday rotation in the high magnetic field regime. (a) Faraday rotation spectra in the high magnetic field regime up to 7 T at 5 K for the sample withEF=60 meV. (b) The magnetic field dependence of the Faraday rotation angle at the photon energy of 4 meV (1 THz). Dashed curve is calculated by the Drude model multiplied by a reduction factor of 0.7 (see text for details). Solid curve is the theoretical calculation obtained from the Kubo formula with the ED method, while dotted curve from the EOM method, both for a phenomenological damping parameterΓ=7 meV. Inset shows the magnetic field dependence of the two LLs in graphene (n=1 and 2) with the green line indicatingEF=60 meV. (c) The EOM calculation for various values ofΓ=5–10 meV (see Methods section for details). (d–f) The same plots asa–c, respectively, for the sample withEF=70 meV. Figure 3: Faraday rotation in the high magnetic field regime. ( a ) Faraday rotation spectra in the high magnetic field regime up to 7 T at 5 K for the sample with E F =60 meV. ( b ) The magnetic field dependence of the Faraday rotation angle at the photon energy of 4 meV (1 THz). Dashed curve is calculated by the Drude model multiplied by a reduction factor of 0.7 (see text for details). Solid curve is the theoretical calculation obtained from the Kubo formula with the ED method, while dotted curve from the EOM method, both for a phenomenological damping parameter Γ =7 meV. Inset shows the magnetic field dependence of the two LLs in graphene ( n =1 and 2) with the green line indicating E F =60 meV. ( c ) The EOM calculation for various values of Γ =5–10 meV (see Methods section for details). ( d – f ) The same plots as a – c , respectively, for the sample with E F =70 meV. Full size image To confirm the origin of the robust plateau structure in the Faraday rotation, let us compare the result with two kinds of theoretical calculations for the optical Hall conductivity, that is, an exact diagonalization (ED) method [10] and an equation of motion (EOM) method [27] (see Method for details). ED, which treats the localization effect, should be accurate in the quantum Hall regime, while it becomes inappropriate, due to the cutoff in the number of included Landau levels, in the classical region for low magnetic fields. EOM method gives a good description for the classical region and a crossover region to the plateau, but gives steeper plateau-to-plateau transitions than the ED method. The results with these complementary methods are plotted in Fig. 3b as solid (ED) and dotted (EOM) curves with multiplying a factor of 0.7 to adjust the absolute value. Although both results have plateau structures, ED result is seen to be closer to the experimental result. To further endorse the correspondence, we plot the result for the Faraday rotation in a sample with E F =70 meV in Fig. 3d . Now, the ν =2 plateau region shifts to higher magnetic fields, while another plateau appears around 3 T. By comparing the LLs and the Fermi energy (inset of Fig. 3e ), the new plateau can be assigned to ν =6, next in the graphene QHE sequence. Correspondingly, the value of the Faraday rotation on this plateau exhibits about three times as large as that for ν =2. The result exhibits an excellent agreement with the numerical calculation (solid curve) for both of the plateaus. Magneto-optical Kerr effect Having seen the robust quantum Hall plateaus in the Faraday rotation, let us now turn to the magneto-optical Kerr effect in a reflection geometry. As shown in Fig. 4a , the short probe pulse used in the THz-TDS enabled us to detect a delayed second pulse that is multiply reflected inside the substrate after the first main pulse with a separation Δt =2 n sub L / c in time-domain, where L is the thickness of the substrate and c the speed of light. The second pulse experiences the Kerr rotation when it reflects at the interface between the substrate and graphene, while experiences the Faraday effect when it transmits graphene, a geometry which has also been adopted to topological insulators [28] , [29] . In the small signal limit ( θ F ( ω ), η F ( ω )<<1), the total rotation angle amounts to the sum of the Faraday and Kerr rotations. Thus, we can extract the Kerr rotation from the delayed second pulse by subtracting the Faraday rotation determined from the polarization of the first pulse. The inset of Fig. 4c shows the Kerr rotation spectra thus obtained for E F =70 meV. 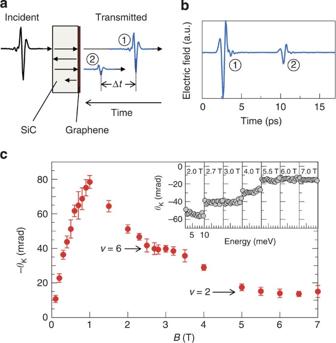Figure 4: Magneto-optical Kerr rotation in the monolayer graphene. (a) Schematic of the transmission of the THz pulse in the sample. (b) The time-domain waveform of the THz pulse transmitted through the sample. (c) The magnetic field dependence of the Kerr rotation at 1 THz for the sample withEF=70 meV. The inset shows the Kerr rotation spectrum at the indicated magnetic fields. Figure 4c shows the magnetic field dependence of the Kerr rotation at 1 THz, where the Kerr rotation angle exhibits a pinned value of θ K =−15 mrad independent of the magnetic field above 5.5 T. The Kerr rotation caused by the reflection at the interface between the substrate and the graphene monolayer is given by Figure 4: Magneto-optical Kerr rotation in the monolayer graphene. ( a ) Schematic of the transmission of the THz pulse in the sample. ( b ) The time-domain waveform of the THz pulse transmitted through the sample. ( c ) The magnetic field dependence of the Kerr rotation at 1 THz for the sample with E F =70 meV. The inset shows the Kerr rotation spectrum at the indicated magnetic fields. Full size image where is the complex reflectivity coefficient for right and left circularly polarized light. In the quantum Hall regime ( σ ± ~ ive 2 / h ), the Kerr rotation is reduced to tan θ K ( ω )~−4 ναn sub /( n sub 2 −1) and anticipated to exhibit θ K ( ω )~−21 mrad for ν =2. The observed Kerr rotation angle of θ K =−15 mrad matches well with this theoretical value if one assumes the reduction factor of 0.7 for the effective fine-structure constant discussed above. Now let us discuss possible origins of the factor of 0.7 in the observed Faraday rotation. One possibility for the smaller rotation is the existence of electron-hole puddles [30] , [31] in the monolayer graphene, which results in the reduction of Faraday rotation. However, the carrier density in the puddles has been estimated to be as low as 10 9 cm −2 from the previous transport measurements in similar epitaxial graphene samples embedded in an FET structure [18] . Thus, the electron-hole puddles may not be considered as a plausible origin. The second possibility is the adsorption of water molecules on the surface of graphene. The reduction of the ‘effective’ fine-structure constant has been reported from the transport measurements in graphene covered by a few layers of water molecules [32] . In our experiments, the sample was set in a cryostat filled with He gas, but not in an ultrahigh vacuum condition, so that adsorption of water molecules in monolayer level was unavoidable. The existence of a buffer layer between the SiC substrate and graphene (see also Methods section) may also affect the effective dielectric constant in equation (1) [33] . In addition, Raman images ( Fig. 1b ) indicate that monolayer graphene covers only a part of the total sample area, where the estimated coverage of 0.8 should also reduce the Faraday rotation. Systematic studies, for example, comparing samples with different coverages, will further elucidate the origin of the reduction factor. To conclude, we have demonstrated the plateau structures and quantum steps in the THz frequency Faraday and Kerr effects in the monolayer graphene associated with the half-integer QHE. At each plateau region, the rotation angle indeed exhibits a fine-structure constant-limited value. In the dc Hall measurement a ‘room-temperature QHE’ has been observed in graphene [34] , so in this context the quantum magneto-optical effect may possibly appear even at room temperature and suggests the potential functionality of graphene for optical storage devices highly robust against fluctuations in magnetic field and also for an achromatic polarization rotator with very high accuracy and low dissipations in the THz frequency range. Another interesting extension of the present experiment will be the optical study of the quantum anomalous Hall effect in graphene [35] , [36] . Sample Monolayer epitaxial graphene samples were grown on 6H-SiC(0001) substrates in an infrared rapid thermal annealing chamber. The SiC was annealed at 1,500 °C in H 2 gas to clean the surface and then annealed at 1,750 °C in Ar gas at a pressure of ~100 Torr. Although the Raman image in Fig. 1b indicates the micrometre scale uniformity of monolayer graphene, the existence of bilayer graphene is discerned in the residual area (for example, point B in Fig. 1b ) as depicted by the Raman spectrum specific to the bilayer graphene ( Fig. 1a ). Small patches of bilayer graphene and the buffer layer should also exist in the monolyer-graphene dominant area [19] , although they cannot be resolved by the present Raman imaging with a spatial resolution of 1 μm. Terahertz time-domain spectroscopy We adopt the THz-TDS for the polarization spectroscopy in the THz frequency range. A mode-locked Ti:Sapphire laser with the wavelength of 800 nm, the pulse width of 110 fs and the repetition rate of 76 MHz was used as a light source. THz pulses were emitted from a p -type InAs, which is irradiated by the laser pulses. The waveform of the THz pulse transmitted after the sample was detected by free-space electro-optical sampling with a (110)-oriented ZnTe crystal. The sample was set in a split-type superconducting magnet cryostat. In order to measure the polarization rotation due to the Faraday and Kerr effects, we used free-standing wire-grid polarizers (WGPs). By setting a WGP placed after the sample parallel ( x -) or orthogonal ( y -) to the incident linear ( x -) polarization, we measured the transmitted THz electric fields E x ( t ) and E y ( t ), respectively. From the Fourier components of the THz field, E x ( ω ) and E y ( ω ), the Faraday rotation θ F ( ω ) and the ellipticity η F ( ω ) are obtained through the relation of E y ( ω )/ E x ( ω )=(sin θ F + iη F cos θ F )/(cos θ F − iη F sin θ F ). In the small angle limit, the relation is simplified as E y ( ω )/ E x ( ω )~ θ F ( ω )+ iη F ( ω ). To detect the small Faraday rotation angle, we measured the signals at both the positive and negative magnetic fields as θ F (+ B ) and θ F (− B ), respectively. The subtraction ( θ F (+ B )− θ F (− B ))/2 eliminates the background signal that arises from the imperfectness of the WGP and enables the detection of small Faraday rotation signal (~mrad) from a monolayer graphene. The error bars in Figs 3b , d were determined by the s.d. of the measurements repeated ten times. For further details of polarization spectroscopy based on THz-TDS, see Ikebe and Shimano [37] . Theoretical calculations We performed two theoretical calculations for the optical Hall conductivity σ xy ( ω ), ED and EOM methods. ED directly applies the Kubo formula, into which the wavefunctions in disordered systems obtained with diagonalization are plugged (Equation 1 in Morimoto et al. [10] ), and an ensemble average over impurity configurations is then taken. In the calculation, E F was fixed (to 60 or 70 meV) and the disorder potential was introduced by randomly placed long-range scatterers, where we set the potential depth of scatterers so that the width of the cyclotron resonance becomes 7 meV in the plateau region (see Morimoto et al. [10] for details). ED method should give an accurate description for the plateau region in the high magnetic field regime, as it fully incorporates the Anderson localization effect from which the plateaus originate, but it should become less accurate for low magnetic fields where LLs become dense and the system approaches classical. Namely, a cutoff in the number of included LLs, which we have to introduce in the diagonalization to have finite-dimensional matrices, gives a good approximation for the QHE regime, but is not appropriate for the classical region where LLs become dense. Incidentally, we note that although the calculation is performed for a fixed Fermi energy, a fixed density of electrons gives a similar result for the plateau structure. On the other hand, EOM is developed by Ferreira et al. [27] , where a magneto-optical conductivity is described through EOM of the current density and concisely reproduces an expression with Green’s function calculations [38] . We have adopted the formula given by equation 55 in Ferreira et al. [27] with a phenomenological damping parameter Γ =7 meV ( Fig. 3b ), as the EOM method agrees with the Drude model in low magnetic fields. Although EOM gives a good description for the classical region and a crossover region towards the QHE, the plateau-to-plateau transition is steeper than that of ED calculation, as the method does not take account of localization effects. Even if we adopt other values of Γ in EOM ( Fig. 3c ), the fits are not improved, and the experimental results in the plateau region are indeed better described by the ED method. How to cite this article: Shimano, R. et al. Quantum Faraday and Kerr rotations in graphene. Nat. Commun. 4:1841 doi: 10.1038/ncomms2866 (2013).